The ubiquitin ligase PDZRN3 is required for vascular morphogenesis through Wnt/planar cell polarity signalling Development and stabilization of a vascular plexus requires the coordination of multiple signalling processes. Wnt planar cell polarity (PCP) signalling is critical in vertebrates for diverse morphogenesis events, which coordinate cell orientation within a tissue-specific plane. However, its functional role in vascular morphogenesis is not well understood. Here we identify PDZRN3, an ubiquitin ligase, and report that Pdzrn3 deficiency impairs embryonic angiogenic remodelling and postnatal retinal vascular patterning, with a loss of two-dimensional polarized orientation of the intermediate retinal plexus. Using in vitro and ex vivo Pdzrn3 loss-of-function and gain-of-function experiments, we demonstrate a key role of PDZRN3 in endothelial cell directional and coordinated extension. PDZRN3 ubiquitinates Dishevelled 3 (Dvl3), to promote endocytosis of the Frizzled/Dvl3 complex, for PCP signal transduction. These results highlight the role of PDZRN3 to direct Wnt PCP signalling, and broadly implicate this pathway in the planar orientation and highly branched organization of vascular plexuses. During development or tissue regeneration, vascular growth is a complex process that can be schematically divided in two dynamic steps. First, a highly unstable vascular plexus is developed, with vessels expanding and collapsing at a high rate. Then, the newly formed vascular system is remodelled to ensure the transition towards a stable and functional network [1] . Evolution towards a structured vascular system is characterized by the formation of a three-dimensional (three-dimensional) hierarchically branched and organized vascular network [2] , suggesting that vascular cells or groups of vascular cells, are instructed to be oriented within stable functional tubes. Recently, several groups, including our own, have provided evidence to underscore the importance of Wnt/Frizzled/planar cell polarity (Wnt/PCP) signalling in vascular system morphogenesis and remodelling [3] , [4] . Evidence has previously linked the Wnt canonical pathway to vascular formation. Mutations of Norrin (Ndp), Frizzled4 (Fzd4), Tetraspanin-12 (TSPAN12) or LRP5, led to ocular syndromes, such as exudative vitreoretinopathy [5] , [6] , [7] , [8] , [9] . In ndp , fzd4 , lrp5 and tspa n12 loss-of-function mice, development of the superficial retinal plexus has been shown to be altered, with a lack of the deep and intermediate vascular plexuses [5] , [6] , [10] , [11] , linking the Wnt canonical signalling complex to vascular formation in the retina. However, the role of the non-canonical PCP pathway is not yet well understood during vessel development and the mechanisms by which the endothelial Wnt/PCP pathway regulates vessel morphogenesis remain elusive. The conserved Wnt/PCP signalling is involved in patterning, by instructing cell polarity within a tissue [12] . First observed in insects, where it regulates the orientation of hair on wings and facets on the eye, Fzd/PCP is now known to be involved in regulating gastrulation and sensory cell orientation in vertebrates [13] . PCP signalling controls basic mechanisms including cell migration, axonal guidance, asymmetric cell division, as well as hair and cilia orientation [14] , [15] . PCP signalling in insects and vertebrates shares a core pathway that includes members of the dishevelled (Dvl1–3 members) [16] and fzd gene families, but is distinct from the β-catenin-dependent canonical Wnt pathway [17] . Dvl proteins are the relays between the Fzd receptor and Wnt downstream signalling pathways [18] . To regulate all of these functions, Dvl has to associate with different protein partners and induce PCP signalling cascades that involve activation of c-jun, a hallmark for PCP signalling and the small GTPAses Rho and Rac [19] . Interestingly, among Dvl members, Dvl3 could be an important relay for Wnt/PCP signalling. Indeed, Dvl3 has a unique function compared with that of the other isoforms in analysing genetic Dvl1-3 mutant phenotypes [16] . In vitro studies showed that Dvl3 compared with Dvl1 and Dvl2 potentiated non-canonical Dab2-dependent activity [20] . Recently, our group has identified an important role for Dvl3 in PCP signalling induction in endothelial cells [21] . To further elucidate the molecular mechanisms regulating the activity of Dvl3 in the PCP pathway, we performed a yeast two-hybrid screening to search for novel Dvl3-interacting proteins. Among these we identified the E3 ubiquitin ligase PDZ domain-containing RING finger protein 3 (PDZRN3). Whereas previously published studies have revealed the role of PDZRN3 in skeletal muscle [22] and osteoblast differentiation acting as an inhibitor of Wnt/b catenin signalling [23] , its role in Wnt signalling is poorly understood. We report that PDZRN3 is expressed in endothelium and using a gene-targeting strategy, we explored the in vivo role of Pdzrn3 during angiogenesis. First, we deleted Pdzrn3 during angiogenic gestational steps from E7.5, taking advantage of the inducible Ubc-Cre ERT2 mice. We report that embryos died very early in utero at E11.5, exhibiting defects in large vitelline vessel morphogenesis in the yolk sac, and impairment of embryonic capillary invasion in the placenta leading to severe growth retardation. Next, we showed that conditional deletion of Pdzrn3 in endothelial cells (EC) in neonates induced a defect in branch extension with excessive vessel regression of the superficial retinal vascular plexus (SRVP), and ultimately a global misorientation of polarized capillaries in the intermediate plexus. In vitro and ex vivo gain and loss of Pdzrn3 expression experiments revealed a role of PDZRN3 in EC coordinated extension, polarization and tubular plexus formation. Mechanistically, we present evidence that PDZRN3 acts as a new partner of Dvl3 and could promote Dvl3 ubiquitinylation, to mediate PCP signalling activation in EC. Taken together, our data reveal a novel and crucial role of Wnt PCP signalling via the ubiquitin ligase PDZRN3 during vascular plexus directional extension and planar organization. PDZRN3 gene deletion induces extraembryonic vascular defects A yeast two-hybrid screen was conducted on an 11.5-days post coitus mouse embryonic library, with Dvl3 as bait in which the DIX domain was deleted(Dvl3ΔDIX) as bait. The DIX domain has been shown to favour the canonical pathway over the PCP pathway [24] , [25] , [26] . We identified PDZRN3, an E3 ubiquitin-protein ligase, shown to negatively regulate Wnt signalling during osteoblast differentiation. As it is widely expressed in various adult mouse tissues [22] ( Supplementary Fig. 1 ), we asked whether PDZRN3 was expressed in a common structure, the endothelium. We first performed real-time reverse transcriptase/PCR experiments on distinct mouse and human primary and cultured endothelial cells, and showed that it is expressed at a high level ( Supplementary Fig. 1a–c ). Then we showed that its expression during angiogenic processes co-localized predominantly with CD31+ vessels in E12.5 yolk sac, E14.5 brain and, postnatally at day 7 (P7), in retinal EC and aortic EC, providing support for a potential role during angiogenesis ( Supplementary Fig. 1d ). To investigate the role of PDZRN3 in blood vessel development, we created mice with targeted deletions of Pdzrn3 , by crossing a homozygous LoxP-flanked Pdzrn3 allele with Cre expression driven by Ubc-cre ERT2 , a potent ubiquitous promoter. Pregnant mice were treated daily with tamoxifen injections from E7.5 to E9.5, to inactivate Pdzrn3 during earlier angiogenesis phases. We verified that PDZRN3 expression at E10.5 was significantly reduced in embryonic brain lysates by western blot ( Fig. 1a ). The Ubc-Cre ERT2 + Pdzrn3 f/f genotype had retarded growth from E9.5 and died between E11.5 and E12.5 ( Fig. 1b,c ). In whole-mount, the pattern of vascularization of Ubc-Cre ERT2 ; Pdzrn3 f/f embryos yolk sacs from E9.5 through E10.5 appeared alteredcompared with that in their wild-type littermates, suggesting a defect in circulation ( Fig. 1c ). At E9.5, all Ubc-Cre ERT2 +; Pdzrn3 f/f mutant yolk sacs showed an altered pattern of distribution compared with wild type, associated with an increase of vitelline artery diameter, while at E10.5, disorganization of the vascular network was more apparent suggesting an inability to complete angiogenic remodelling ( Fig. 1c ). It is worth noting that tamoxifen treatment of pregnant mice from E10.5 to E12.5 did not induce lethality ( Fig. 1b ), indicating a key role for Pdzrn3 in the early angiogenic phases. Histological analysis of the placenta from E9.5 and E10.5 mutant embryos revealed that, while chorio-allantoic fusion had occurred, the labyrinth layer was reduced and fetal capillaries invading the labyrinth were absent. Comparatively, in wild-type embryos, fetal vessels were evenly distributed throughout the labyrinth ( Fig. 1d ). Ubc-Cre ERT2 Pdzrn3 f/f embryo vasculature, revealed by whole-mount platelet endothelial cell adhesion molecule staining, appeared altered with reduction of the brain vasculature ( Fig. 1e ). Taken together, our results suggest that severe growth retardation and embryonic death, at mid gestation in Ubc-Cre ERT2 + Pdzrn3 f/f mice, could be caused by defective yolk sac circulation and/or placenta function. 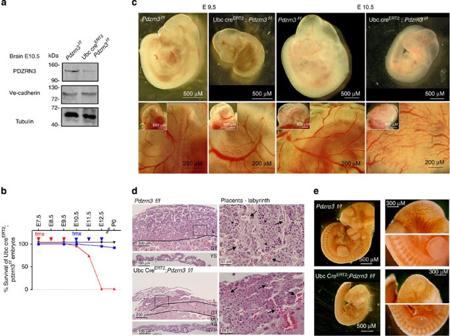Figure 1:UbccreERT2Pdzrn3f/fembryos displayed defects in yolk-sac and placental angiogenesis. (a) Level ofPdzrn3depletion inUbccreERT2Pdzrn3f/fversusPdzrn3f/fmice was evaluated by western blot on E10.5 embryo brain lysates after tamoxifen treatment of pregnant mothers at E7.5. Normalization was done using the expression of α-tubulin. (b) Survival rate ofUbccreERT2Pdzrn3f/fembryos was measured after gene deletion induced by daily tamoxifen treatment (tmx) of pregnant mothers at E7.5 (red arrowhead) (n=214) or at E10.5 (blue arrowhead) (n=44).Pdzrn3deletion at E7.5 leads to growth retardation and early embryo lethality from E11.5 to E12.5 (n=79). (c) Deletion ofPdzrn3-coding gene by tamoxifen injection at E7.5 leads to severe growth retardation as observed at E9.5 and E10.5.UbccreERT2Pdzrn3f/fembryos were significantly smaller and exhibited abnormal vascularization of the yolk sac (scale bar, 500 μm). Whole-mount visualization ofUbccreERT2Pdzrn3f/fversusPdzrn3f/fyolk sac demonstrated an organized and ordered vitelline architecture in control mice, while this network was disorganized in mutant embryos at E9.5 and E10.5. Scale bar, 500 μm in the inset and 200 μm at a higher magnification. (d) Placental vasculature was examined in haematoxylin/eosin-stained sections of control and mutant placentas at E9.5, revealing a reduced labyrinth layer inUbccreERT2Pdzrn3f/fmutant embryos (scale bar, 100 μm). In a higher magnification, embryonic vessels (arrowhead), as defined by the presence of nucleated red cells are evenly distributed in the labyrinth inPdzrn3f/fcontrol placenta while in mutant placentas they are missing (scale bar, 50 μm). Embryonic vessels are close to maternal vessels (arrow) in control embryos, indicating that maternal–fetal exchanges occur in control but not in mutant embryos. MD: maternal deciduas; GT: giant trophoblasts; L: labyrinth; YS: yolk sac. (e) Whole-mount of CD31 ofUbccreERT2Pdzrn3f/fmutant andPdzrn3f/fcontrol embryos. Vessel network of the brain, but not of the somites is altered in mutants compared with controls at E10.5 (scale bar, 500 μm; 300 μm in insets). The mutant embryo showed fewer vessels and branches in the brain. Figure 1: Ubc creERT2 Pdzrn3 f/f embryos displayed defects in yolk-sac and placental angiogenesis. ( a ) Level of Pdzrn3 depletion in Ubc creERT2 Pdzrn3 f/f versus Pdzrn3 f/f mice was evaluated by western blot on E10.5 embryo brain lysates after tamoxifen treatment of pregnant mothers at E7.5. Normalization was done using the expression of α-tubulin. ( b ) Survival rate of Ubc creERT2 Pdzrn3 f/f embryos was measured after gene deletion induced by daily tamoxifen treatment (tmx) of pregnant mothers at E7.5 (red arrowhead) ( n =214) or at E10.5 (blue arrowhead) ( n =44). Pdzrn3 deletion at E7.5 leads to growth retardation and early embryo lethality from E11.5 to E12.5 ( n =79). ( c ) Deletion of Pdzrn3 -coding gene by tamoxifen injection at E7.5 leads to severe growth retardation as observed at E9.5 and E10.5. Ubc creERT2 Pdzrn3 f/f embryos were significantly smaller and exhibited abnormal vascularization of the yolk sac (scale bar, 500 μm). Whole-mount visualization of Ubc creERT2 Pdzrn3 f/f versus Pdzrn3 f/f yolk sac demonstrated an organized and ordered vitelline architecture in control mice, while this network was disorganized in mutant embryos at E9.5 and E10.5. Scale bar, 500 μm in the inset and 200 μm at a higher magnification. ( d ) Placental vasculature was examined in haematoxylin/eosin-stained sections of control and mutant placentas at E9.5, revealing a reduced labyrinth layer in Ubc creERT2 Pdzrn3 f/f mutant embryos (scale bar, 100 μm). In a higher magnification, embryonic vessels (arrowhead), as defined by the presence of nucleated red cells are evenly distributed in the labyrinth in Pdzrn3 f/f control placenta while in mutant placentas they are missing (scale bar, 50 μm). Embryonic vessels are close to maternal vessels (arrow) in control embryos, indicating that maternal–fetal exchanges occur in control but not in mutant embryos. MD: maternal deciduas; GT: giant trophoblasts; L: labyrinth; YS: yolk sac. ( e ) Whole-mount of CD31 of Ubc creERT2 Pdzrn3 f/f mutant and Pdzrn3 f/f control embryos. Vessel network of the brain, but not of the somites is altered in mutants compared with controls at E10.5 (scale bar, 500 μm; 300 μm in insets). The mutant embryo showed fewer vessels and branches in the brain. Full size image Furthermore, we created mice with targeted deletions of Pdzrn3, by crossing a LoxP-flanked Pdzrn3 gene with Cre expression driven by a Pdgf tamoxifen-inducible promoter, which targets ECs [68] . We then analysed Pdgf icre Pdzrn3 f/f embryo mutants (iEC knockout (KO)) between E9.5 and E11.5 versus Pdzrn3f/f embryo controls (iEC wild type (WT)) ( Supplementary Fig. 2 ). We observed an altered pattern of vessel organization in the yolk sacs of the iEC KO embryos similar to that reported for the Ubc-CreERT2+Pdzrn3f/f mutants ( Supplementary Fig. 2a ). Moreover, histological analysis of mutant placenta at E10.5 revealed a statistical decrease in the number of embryonic vessels that invade the labyrinth layer ( Supplementary Fig. 2b ). However, it is noteworthy that the alterations of the embryo vascular network, either in yolk sacs or placenta, were milder than the one found under Ubc-Cre ERT2 depletion and only 25% of the iEC KO embryos had growth retarded at E11.5. This less-severe phenotype may be due to an incomplete cre-mediated excision of Pdzrn3 or linked to Pdzrn3 role in non-endothelial cells. In conclusion, this complementary genetic approach strongly supports a direct role for Pdzrn3 on vascular yolk sac organization and the development of the embryonic vascular labyrinth structure in placenta. PDZRN3 gene deletion in ECs induces vascular defects Next, we analysed the effects of PDZRN3 deficiency on vessel morphogenesis postnatally, in the mouse retina. Western blots on wild-type whole-retinal lysates from P3 to P21 showed that PDZRN3 is expressed in EC, with peak expression at P12, which coincides with intense vascular remodelling ( Fig. 2a ). Postnatal recombination efficiency was evaluated by crossing mT/mG Pdzrn3 f/f reporter mice with Pdgf icre +Pdzrn3 f/f mice. Depletion of Pdzrn3 was verified by western blot in Pdzrn3 iECKO versus littermate control ( Pdzrn3 iECWT ) retina lysates ( Fig. 2b ). Retina from Pdzrn3 iECKO mice had delayed vascularization of the SRVP at P5 ( Supplementary Fig. 3 ) and P7 compared with control Pdzrn3 iECWT mice, with reduced vascular density and a decrease in the number of branch points, while EC proliferation was significantly increased in tip cells and in the plexus as revealed after BrdU injection. Pdzrn3 iECKO vessels appeared to be unstable, with an increase in the number of empty collagen IV-positive/isolectin-B4-negative ‘sleeves’ in the central areas ( Fig. 2c ). The number of tip cells was not affected. At P12, the SVRP still displayed excessive capillary regression ( Fig. 2d ). Interestingly, in control retinas the deep capillary plexus displayed a complex hexagonal pattern, reminiscent of honeycomb structures, while in mutant retinas the capillary network was abnormal and massively reduced. To test whether Pdzrn3 deletion could alter plexus formation via the PCP pathway, we analysed the planar polarized organization of the intermediate capillary network, which forms bridges between the parent apical plexus (SRVP) and the parallel basal deep plexus (deep retinal vascular plexus). This intermediate network emerged in a two-dimensional sheet, orthogonal to the axis of the SRVP ( Fig. 2d ). We collected confocal images and extracted capillary skeletons in this plane, which revealed that the pattern of vessel organization from SRVP to deep retinal vascular plexus was altered. In mutants, capillaries that initiated from the SRVP subsequently pointed in inappropriate directions in the deepest plexus compared with that of the well-organized polarized network in control mice ( Fig. 2e ). These data demonstrate that Pdzrn3 deletion alters vessel remodelling and stabilization during retinal angiogenesis, and impairs polarized capillary structure formation during tertiary plexus formation. 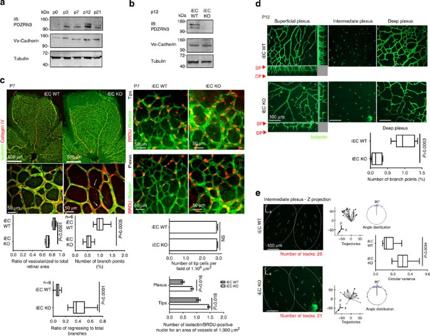Figure 2: PDZRN3 is essential in EC for capillary extension/stabilization and 2D directional angiogenesis during retina vascular development. (a) Wild-type retina protein extracts, evaluated by western blot, revealed that PDZRN3 levels peak at P12; normalization was done using Ve-cadherin and α-tubulin. (b) Postnatal tamoxifen treatment induced PDZRN3 ablation inPdzrn3iECKO(iEC KO) versusPdzrn3iECWT(iEC WT) retinal protein extracts at P12. Normalization was done using Ve-cadherin and α-tubulin. (c) Confocal images of retina showing a reduced area of vascularization, of the number of branch points in iEC KO versus iEC WT retinal vasculature at P7 and an increase in regressing isolectin-B4−/collagen IV+branches (arrow). Scale bars, 500 μm and 50 μm in upper and lower panels, respectively. Proliferation is increased in iEC KO versus iEC WT vasculature in both tip and plexus areas as indicated by quantification of BrdU- (red) isolectin-B4- (green) positive nuclei related to the vessel surface. The error bars represent mean and s.d.n=6 for iEC KO;n=6 for iEC WT. Unpairedt-test. Scale bars, 50 μM. (d) At P12, formation of the intermediate and deep plexus is altered inPdzrn3iECKOcompared with that inPdzrn3iECWTmice. The number of branch points after isolectin-B4 (green) staining in the deep plexus was decreased from iEC KO versus iEC WT. The intermediate plexus is severely disorganized in iEC KO mice. Transverse reconstruction of retinal images obtained by confocal microscopy shows the intermediate plexus organization linking the superficial (SP) to the deep (DP) retinal vascular plexus in a 2D orthogonal plane. The error bars represent mean and s.d.n=6 for iEC KO;n=6 for iEC WT. Unpairedt-test. Scale bar, 100 μm. (e) Three-dimensional projected Z-stacks views of the intermediate plexus revealed a disorganization of the plexus capillary network when retinas from iEC KO are compared with iEC WT retinas. The orientation of the branches of the intermediate plexus was represented by vectors indicating their direction between two Z planes in thexandyaxis planes. Scale bar, 100 μm. Circular variance indicates how much orientations deviate from the mean.n=10 iEC KO; 10 iEC WT. Unpairedt-test. Figure 2: PDZRN3 is essential in EC for capillary extension/stabilization and 2D directional angiogenesis during retina vascular development. ( a ) Wild-type retina protein extracts, evaluated by western blot, revealed that PDZRN3 levels peak at P12; normalization was done using Ve-cadherin and α-tubulin. ( b ) Postnatal tamoxifen treatment induced PDZRN3 ablation in Pdzrn3 iECKO (iEC KO) versus Pdzrn3 iECWT (iEC WT) retinal protein extracts at P12. Normalization was done using Ve-cadherin and α-tubulin. ( c ) Confocal images of retina showing a reduced area of vascularization, of the number of branch points in iEC KO versus iEC WT retinal vasculature at P7 and an increase in regressing isolectin-B4 − /collagen IV + branches (arrow). Scale bars, 500 μm and 50 μm in upper and lower panels, respectively. Proliferation is increased in iEC KO versus iEC WT vasculature in both tip and plexus areas as indicated by quantification of BrdU- (red) isolectin-B4- (green) positive nuclei related to the vessel surface. The error bars represent mean and s.d. n =6 for iEC KO; n =6 for iEC WT. Unpaired t -test. Scale bars, 50 μM. ( d ) At P12, formation of the intermediate and deep plexus is altered in Pdzrn3 iECKO compared with that in Pdzrn3 iECWT mice. The number of branch points after isolectin-B4 (green) staining in the deep plexus was decreased from iEC KO versus iEC WT. The intermediate plexus is severely disorganized in iEC KO mice. Transverse reconstruction of retinal images obtained by confocal microscopy shows the intermediate plexus organization linking the superficial (SP) to the deep (DP) retinal vascular plexus in a 2D orthogonal plane. The error bars represent mean and s.d. n =6 for iEC KO; n =6 for iEC WT. Unpaired t -test. Scale bar, 100 μm. ( e ) Three-dimensional projected Z-stacks views of the intermediate plexus revealed a disorganization of the plexus capillary network when retinas from iEC KO are compared with iEC WT retinas. The orientation of the branches of the intermediate plexus was represented by vectors indicating their direction between two Z planes in the x and y axis planes. Scale bar, 100 μm. Circular variance indicates how much orientations deviate from the mean. n =10 iEC KO; 10 iEC WT. Unpaired t -test. Full size image PDZRN3 knock down modulates EC migration and sprout regression We then explored whether the observed angiogenic phenotype in Pdzrn3 mutants was due to EC motility defects. First, we analysed the role of PDZRN3 on EC migration under Wnt induction. Cell tracking of migrating EC revealed that Wnt5a enhanced the distance of EC migration compared with control conditions ( Fig. 3a ). We then showed that Pdzrn3 depletion, using small interfering RNA (siRNA), impairs Wnt5a-induced EC migration and that conversely, lentiviral Pdzrn3 transduction markedly enhanced EC migration in Wnt5a-treated conditions. Importantly, Pdzrn3 -depleted cells lost their ability to migrate in a directional manner while Pdzrn3 lentivirus-transduced EC migrated primarily in a straight path, in Wnt5a conditions ( Fig. 3a ). 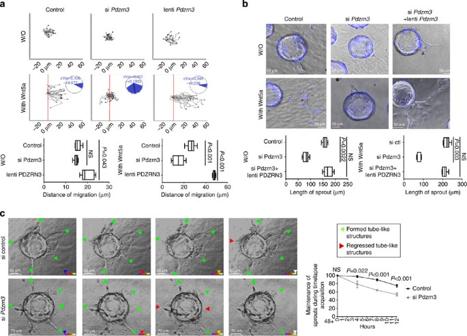Figure 3: PDZRN3 regulates EC migration and tube formation in a Wnt5a-dependent manner. (a) PDZRN3 regulates migration of HUVEC under Wnt5a activation. Migration is repressed after siPdzrn3treatment and activated afterPdzrn3transduction (lenti Pdzrn3). The migration distance was followed by time laps and calculated based upon recorded images taken 6 h after Wnt5a activation for 10 h; quantification is provided in the graph. Migration plot analysis shows the direction of migration of EC. Quantification of the distance of migration using Imaris is shown. Circular variance indicates how much the orientation deviates from the directional mean. Experiments were performed in triplicate, error bars denote s.d.,n=3; unpairedt-test on average measure of three independent experiments—~20 tracks analysed per field. (b) PDZRN3 regulates three-dimensional (3D) tubulogenesis of HUVEC. A suspension of HUVEC-coated cytodex beads were embedded in fibrin gels, in the presence of fibroblasts transfected to express Wnt5a (with Wnt5a) or not (W/O). Nuclei were stained with Hoechst dye and images were acquired 96 h after plating. For each experiment, sprout length after 96 h was measured. In the presence of Wnt5a, sprout formation was enhanced. siPdzrn3-treated HUVEC exhibited impaired sprout formation as compared with control-treated HUVEC in both W/O or with Wnt5a conditions. Transduction ofPdzrn3was able to reversePdzrn3siRNA impairment of sprout formation and response to Wnt5a. Experiments performed in triplicate, bars denote min to max,n=3, five beads were analysed per condition. Unpairedt-test on the average values obtained in three independent experiments. Scale bars, 50 μM. (c)Pdzrn3regulates stability of tube-like structures in the 3D tubulogenesis assay. The cytodex preparation was subjected to time-lapse imaging between 48 (48H+T0H) and 64 (48H+T16H) hours after plating with an acquisition each 30 min. In control conditions, the majority of sprouts were stable and extending (green arrows) during the whole acquisition (16 h) while inPdzrn3-depleted conditions, most of the sprouts were unstable, as indicated by the large number of regressing sprouts (red arrows). Scale bars, 50 μm The number of stable sprouts at the different time points was quantified. Experiments performed in triplicate, bars denote s.d.,n=3, five beads were analysed per condition. Unpairedt-test on the average values obtained in three independent experiments. NS, not significant. Figure 3: PDZRN3 regulates EC migration and tube formation in a Wnt5a-dependent manner. ( a ) PDZRN3 regulates migration of HUVEC under Wnt5a activation. Migration is repressed after si Pdzrn3 treatment and activated after Pdzrn3 transduction ( lenti Pdzrn3 ). The migration distance was followed by time laps and calculated based upon recorded images taken 6 h after Wnt5a activation for 10 h; quantification is provided in the graph. Migration plot analysis shows the direction of migration of EC. Quantification of the distance of migration using Imaris is shown. Circular variance indicates how much the orientation deviates from the directional mean. Experiments were performed in triplicate, error bars denote s.d., n =3; unpaired t -test on average measure of three independent experiments—~20 tracks analysed per field. ( b ) PDZRN3 regulates three-dimensional (3D) tubulogenesis of HUVEC. A suspension of HUVEC-coated cytodex beads were embedded in fibrin gels, in the presence of fibroblasts transfected to express Wnt5a (with Wnt5a) or not (W/O). Nuclei were stained with Hoechst dye and images were acquired 96 h after plating. For each experiment, sprout length after 96 h was measured. In the presence of Wnt5a, sprout formation was enhanced. si Pdzrn3- treated HUVEC exhibited impaired sprout formation as compared with control-treated HUVEC in both W/O or with Wnt5a conditions. Transduction of Pdzrn3 was able to reverse Pdzrn3 siRNA impairment of sprout formation and response to Wnt5a. Experiments performed in triplicate, bars denote min to max, n =3, five beads were analysed per condition. Unpaired t -test on the average values obtained in three independent experiments. Scale bars, 50 μM. ( c ) Pdzrn3 regulates stability of tube-like structures in the 3D tubulogenesis assay. The cytodex preparation was subjected to time-lapse imaging between 48 (48H+T0H) and 64 (48H+T16H) hours after plating with an acquisition each 30 min. In control conditions, the majority of sprouts were stable and extending (green arrows) during the whole acquisition (16 h) while in Pdzrn3- depleted conditions, most of the sprouts were unstable, as indicated by the large number of regressing sprouts (red arrows). Scale bars, 50 μm The number of stable sprouts at the different time points was quantified. Experiments performed in triplicate, bars denote s.d., n =3, five beads were analysed per condition. Unpaired t -test on the average values obtained in three independent experiments. NS, not significant. Full size image Next, we assessed whether PDZRN3 is required for sprouting extension using an assay for collective EC migration, where Human umbilical vein endothelial cells (HUVECs) form sprouts in a fibrin gel ( Fig. 3b ). In this assay, we first confirmed that Wnt5a enhanced angiogenic sprout lengths, by showing that Wnt5a-transfected fibroblasts layered on top of the gel enhanced EC tube length significantly, compared with control fibroblasts. Ninety-six hours after plating, silencing of Pdzrn3 blocked cells from leaving the beads in response to basal or Wnt5a conditions. Pdzrn3 -silenced EC did not migrate collectively and could not form long, multi-nuclei branched structures, while PDZRN3 lentiviral transdution of Pdzrn3 -silenced HUVECs restored 3D EC migration in response to basal or Wnt5a conditions ( Fig. 3b ). The analysis of the duration of a tube-like structure on recorded time-lapse images revealed that sprouts are dynamically formed over the course of 16 h, while Pdzrn3 -silenced EC were incapable of maintaining sprouts. These data demonstrate the role of PDZRN3 in favouring capillary-like structure formation and stabilization ( Fig. 3c ). Pdzrn3 regulates Dvl3 ubiquitinylation We then explored mechanistically, the role of PDZRN3 in endothelial morphogenetic events. First, we confirmed that at endogeneous levels Dvl interacts with PDZRN3. In Pdzrn3 iECWT lung lysates, co-immunoprecipitation of endogenous Dvl3 using anti-Dvl3 antibody, co-precipitated PDZRN3, which included several ubiquitin chains, whereas in Pdzrn3 iECKO lung extracts, the Dvl3-PDZRN3 interactions and Dvl3 ubiquitinylation were markedly reduced ( Fig. 4a ). 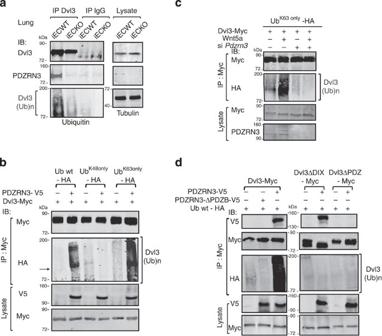Figure 4: PDZRN3 regulates Dvl3 ubiquitinylation. (a) Dvl3 ubiquitinylation required PDZRN3 activity. Lung homogenates fromPdzrn3iECKO(iEC KO) compared with that inPdzrn3iECWTmice versus (iECWT) mice were subjected to immunoprecipitation with anti-Dvl3 or non-immune (IgG) antibodies, followed by anti-PDZRN3 and anti-ubiquitin immunoblotting. (b) PDZRN3 induces Dvl3 ubiquitinylation preferentially with K63-dependent ubiquitin chains. Ubiquitinylation of Dvl3 is induced in HEK293 cells transfected with PDZRN3-V5 in the presence of either UB wt-HA or UBK63only-HA, but not in the presence of UBK48only-HA. (c) PDZRN3 ubiquitinylates Dvl3 in a Wnt-dependent manner. Depletion ofPdzrn3in HeLa cells (siPdzrn3) inhibits UbK63-dependent ubiquitinylation of Dvl3 induced by Wnt5a CM. Ubiquitinylation of the Dvl3 is indicated by co-precipitation of Dvl3-Myc with HA-tagged polyubiquitin chains. Western blot uncropped scans are shown inSupplementary Fig. 5. (d) Co-precipitation of Dvl3 and PDZRN3 requires the PDZ domain of Dvl3 and the PDZB (PDZ binding) domain of PDZRN3. PDZRN3-V5, but not PDZRN3ΔPDZB-V5, induces co-precipitation of Dvl3-Myc; PDZRN3-V5 cannot co-precipitate Dvl3ΔPDZ-Myc. PDZRN3-V5 induces co-precipitation of Dvl3-Myc, but not Dvl3ΔDIX-Myc, with HA-tagged polyubiquitin chains, suggesting that the DIX domain of Dvl3 is required for ubiquitinylation by PDZRN3. Figure 4: PDZRN3 regulates Dvl3 ubiquitinylation. ( a ) Dvl3 ubiquitinylation required PDZRN3 activity. Lung homogenates from Pdzrn3 iECKO (iEC KO) compared with that in Pdzrn3 iECWT mice versus (iECWT) mice were subjected to immunoprecipitation with anti-Dvl3 or non-immune (IgG) antibodies, followed by anti-PDZRN3 and anti-ubiquitin immunoblotting. ( b ) PDZRN3 induces Dvl3 ubiquitinylation preferentially with K63-dependent ubiquitin chains. Ubiquitinylation of Dvl3 is induced in HEK293 cells transfected with PDZRN3-V5 in the presence of either UB wt-HA or UB K63only -HA, but not in the presence of UB K48only -HA. ( c ) PDZRN3 ubiquitinylates Dvl3 in a Wnt-dependent manner. Depletion of Pdzrn3 in HeLa cells (si Pdzrn3 ) inhibits Ub K63 -dependent ubiquitinylation of Dvl3 induced by Wnt5a CM. Ubiquitinylation of the Dvl3 is indicated by co-precipitation of Dvl3-Myc with HA-tagged polyubiquitin chains. Western blot uncropped scans are shown in Supplementary Fig. 5 . ( d ) Co-precipitation of Dvl3 and PDZRN3 requires the PDZ domain of Dvl3 and the PDZB (PDZ binding) domain of PDZRN3. PDZRN3-V5, but not PDZRN3ΔPDZB-V5, induces co-precipitation of Dvl3-Myc; PDZRN3-V5 cannot co-precipitate Dvl3ΔPDZ-Myc. PDZRN3-V5 induces co-precipitation of Dvl3-Myc, but not Dvl3ΔDIX-Myc, with HA-tagged polyubiquitin chains, suggesting that the DIX domain of Dvl3 is required for ubiquitinylation by PDZRN3. Full size image We further investigated whether Dvl3 was a substrate of PDZRN3-mediated ubiquitinylation. We co-expressed either Ub WT-haemagglutinin (HA) or Ub K48only -HA and Ub K63only -HA, in which all the lysine residues are mutated to arginine, except Lys48 or Lys63, respectively, with Dvl3-myc. PDZRN3-V5 was able to induce Dvl3 ubiquitinylation in the presence of either Ub WT-HA or Ub K63only -HA, but not with HA-Ub K48only . As Lys63 is the major site for PDZRN3-mediated polyubiquitinylation of Dvl3, our data suggest that ubiquitinylation of Dvl3 by PDZRN3 is an intracellular signal promoting Dvl3 trafficking ( Fig. 4b ). Since Dvl proteins are known to be involved in endocytosis during Wnt/PCP signalling [27] , [28] , [29] , [30] , we hypothesized that PDZRN3 may facilitate endocytosis of the Dvl3 complex, to induce non-canonical PCP signalling. To test this hypothesis, we followed Dvl3 ubiquitinylation under Wnt/PCP activation. Incubation with Wnt5a conditioned medium (CM) for 1 h induced ubiquitinylation of Dvl3-Myc in HEK293T cells co-transfected with Ub K63only -HA and Dvl3-Myc ( Fig. 4c ). However, Wnt5a failed to induce Dvl3-Myc ubiquitinylation in Pdzrn3 -depleted cells using siRNA. These results demonstrate that PDZRN3 is required for Wnt5a-mediated ubiquinylation of Dvl3-Myc. To understand how Dvl3 interacts with PDZRN3, we sought to identify the domains in Dvl3 and PDZRN3 that are important for their interaction and for PDZRN3 ubiquitinylation activity ( Fig. 4d ). When PDZRN3-V5 was co-transfected with Dvl3-myc and HA-tagged Ubiquitin (Ub Wt-HA) in HeLa cells, Dvl3 ubiquitinylation was detected as a smear of bands in the anti-myc immunoprecipitate with anti-HA. Interestingly, PDZRN3 could not induce ubiquitinylation of Dvl3ΔDIX in the presence of Ub-HA, suggesting that PDZRN3 ubiquitinylates Dvl3 on its DIX domain. We identified the domains of PDZRN3 required for interaction with Dvl3. As the Thr-Thr-Val-COOH motif (TTV motif) has previously been characterized as a PDZ-binding domain (PDZB) [31] , [32] , we co-expressed Dvl3-myc with PDZRN3 deleted from the C-terminal TTV motif (PDZRN3ΔPDZB). Dvl3-myc was unable to precipitate PDZRN3ΔPDZB, demonstrating that the PDZ-binding motif (TTV) of PDZRN3 is required for PDZRN3 binding to Dvl3. Next, we mapped the PDZRN3-interacting domain of Dvl3 using various myc-tagged Dvl3 constructs [21] . Deletion of PDZ (Dvl3ΔPDZ), but not the DIX (Dvl3ΔDIX) domain, impaired Dvl3 immunoprecipitation of PDZRN3 ( Fig. 4d ). These data show that the interaction between PDZRN3 and Dvl3 is mediated by the C-terminal PDZRN3 PDZ-binding domain and the PDZ domain of Dvl3. Pdzrn3 silencing impairs Frizzled/Dvl3 endocytosis We previously demonstrated that Fzd4 recruits Dvl3 at the cell membrane to induce PCP signalling. Here we analysed whether PDZRN3 could be recruited to the Fzd4/Dvl3 complex at the cell membrane. Examination of subcellular distribution of the three partners (PDZRN3, Fzd4 and Dvl3) showed that in Fzd4-HA-transfected HeLa cells, PDZRN3-V5 and Dvl3-Myc re-localized from the cytoplasm to the cell membrane, co-localizing with Fzd4-HA ( Supplementary Fig. 4 ). In the presence of Dvl3ΔPDZ-Myc and PDZRN3-V5, only Dvl3ΔPDZ-Myc was re-localized to the cell membrane with Fzd4-HA, while PDZRN3-V5 stayed in the cytoplasm ( Supplementary Fig. 4 ). This result supports the notion that the interaction between PDZRN3 and Dvl3, via the PDZ domain of Dvl3, is required for recruitment of PDZRN3 towards Fzd4. Next, we examined the role of PDZRN3 in endocytosis of the Fzd4/Dvl3 complex upon activation of Wnt5a, using in vitro models. Immunoprecipitation assays demonstrated that Wnt5a treatment induces Fzd4/Dvl3 re-localization in the Rab5-positive compartment, and its effects are impaired under conditions of Pdznr3 depletion ( Fig. 5a ). Using cell-fractionation approaches, we confirmed that Wnt5a treatment induces re-localization of the Fzd4/Dvl3 complex from the cytosolic membrane to early-endosome fractions. Treatment with either the inhibitor of dynamin, dynasore, or depletion of Pdzrn3 , blocked Fzd4/Dvl3 re-localization ( Fig. 5b ). Using confocal imaging, we next demonstrated that Fzd4 accumulates at the cell membrane in HeLa cells transiently transfected with HA-tagged Fzd4, while 30 min of exposure to Wnt5a induces re-localization of Fzd4 in the intracellular compartment. PDZRN3 is required for the process, as internalization of Fzd4 was efficiently blocked when Pdzrn3 was depleted with siRNA ( Fig. 5c ). Fzd4 was detected in intracellular Rab5-positive early-endosome vesicles after incubation with Wnt5a CM, as shown by an overlapping punctate staining pattern of HA-Fzd4 with Rab5. Pdzrn3 depletion via siRNA transfection or treatment with the inhibitor of dynamin, dynasore, abolished Fzd4 co-localization with Rab5 in intracellular cargos under Wnt5a activation. Co-localization of Fzd4 with Rab5 was quantified in each condition ( Fig. 5c ). 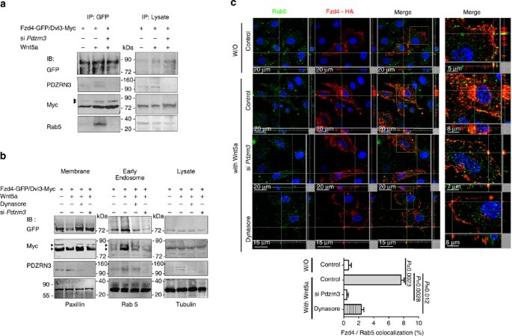Figure 5: PDZRN3 is required for Fzd4 endocytosis upon Wnt5a activation. (a) PDZRN3 is required for Wnt5a-mediated internalization of Fzd4, as indicated by co-precipitation of Fzd4-GFP and Dvl3-myc with Rab5 in HEK293 cells after incubation with Wnt5a CM, but not in siPdzrn3-treated cells. Wnt5a treatment induces co-precipitation of Fzd4 and Dvl3 in a phosphorylated (activated) form, as indicated by the shift of mobility (arrowhead). (b) Wnt5a induces recruitment of Fzd4-GFP and Dvl3 to the early-endosome fraction in a PDZRN3-dependent manner. In HeLa cells, transfected Fzd4-GFP and Dvl3-myc are detected mostly in the membrane fraction. After Wnt5a treatment, levels of Fzd4-GFP and Dvl3 are reduced in the membrane fraction, and are partially relocated to the early-endosome fraction. Treatment with an endocytosis inhibitor, dynasore, or with siPdzrn3, blocks Wnt5a-mediated Fzd4/Dvl3 recruitment to the endosome. The membrane fraction was normalized using paxillin; the early endosome using Rab5 and the lysate with tubulin. Western blot uncropped scans are shown inSupplementary Fig. 5. (c) Depletion ofPdzrn3in HeLa cells inhibits Wnt5a-dependent re-localization of Fzd4 to Rab5-positive vesicles. Immunofluorescence analysis detected Rab5 (green) in cytoplasmic vesicles and Fzd4-HA (red) at the cell membrane in control CM-treated cells (W/O, control). Merged image of Fzd4-HA and Rab5 and magnification view of insets shows that Fzd4 is relocated to Rab5-positive cytoplasmic punctates in HeLa cells exposed to Wnt5a CM treatment as indicated by co-localization (yellow) but not inPdzrn3-depleted cell (siPdzrn3) or those treated with dynasore. Scale bar, 20 μm. Experiments were performed in triplicate; bars denote min to max,n=3. Unpairedt-test on the average values obtained in three independent experiments. Figure 5: PDZRN3 is required for Fzd4 endocytosis upon Wnt5a activation. ( a ) PDZRN3 is required for Wnt5a-mediated internalization of Fzd4, as indicated by co-precipitation of Fzd4-GFP and Dvl3-myc with Rab5 in HEK293 cells after incubation with Wnt5a CM, but not in si Pdzrn3 -treated cells. Wnt5a treatment induces co-precipitation of Fzd4 and Dvl3 in a phosphorylated (activated) form, as indicated by the shift of mobility (arrowhead). ( b ) Wnt5a induces recruitment of Fzd4-GFP and Dvl3 to the early-endosome fraction in a PDZRN3-dependent manner. In HeLa cells, transfected Fzd4-GFP and Dvl3-myc are detected mostly in the membrane fraction. After Wnt5a treatment, levels of Fzd4-GFP and Dvl3 are reduced in the membrane fraction, and are partially relocated to the early-endosome fraction. Treatment with an endocytosis inhibitor, dynasore, or with si Pdzrn3 , blocks Wnt5a-mediated Fzd4/Dvl3 recruitment to the endosome. The membrane fraction was normalized using paxillin; the early endosome using Rab5 and the lysate with tubulin. Western blot uncropped scans are shown in Supplementary Fig. 5 . ( c ) Depletion of Pdzrn3 in HeLa cells inhibits Wnt5a-dependent re-localization of Fzd4 to Rab5-positive vesicles. Immunofluorescence analysis detected Rab5 (green) in cytoplasmic vesicles and Fzd4-HA (red) at the cell membrane in control CM-treated cells (W/O, control). Merged image of Fzd4-HA and Rab5 and magnification view of insets shows that Fzd4 is relocated to Rab5-positive cytoplasmic punctates in HeLa cells exposed to Wnt5a CM treatment as indicated by co-localization (yellow) but not in Pdzrn3- depleted cell (si Pdzrn3 ) or those treated with dynasore. Scale bar, 20 μm. Experiments were performed in triplicate; bars denote min to max, n =3. Unpaired t -test on the average values obtained in three independent experiments. Full size image PDZRN3 favours non-canonical Wnt/PCP pathway We investigated whether PDZRN3 could regulate the Wnt signalling pathway using western blot. We evaluated active β-catenin (ABC) and p–c-jun levels as markers of canonical and PCP Wnt pathways, respectively ( Fig. 6a ). There was significant upregulation of ABC expression with a downregulation of p–c-jun in EC isolated from Pdzrn3 iECWT versus Pdzrn3 iECKO lungs at P7, suggesting that PDZRN3 is required to attenuate the Wnt/β catenin canonical signal transduction and to promote the Wnt/PCP pathway in postnatal EC, confirming previous work on cultured osteoblast differentiation [23] . To test this hypothesis, we followed β-catenin activation in cultured EC under Wnt3a activation. Our data showed that, under basal conditions and after Wnt3a stimulation, β-catenin and ABC expression were significantly elevated in Pdzrn3- depleted EC versus control EC ( Fig. 6b ). Interestingly, upregulation of p–c jun by Wnt5a was impaired in Pdzrn3 -depleted cells ( Fig. 6c ). Next, β-catenin transcriptional activity was measured using the Top-Flash/luciferase reporter construct. Again, we observed that under basal conditions and after Wnt3a stimulation, the Top flash reporter was more robustly activated in EC depleted of Pdzrn3 with siRNA versus control, and reduced in Pdzrn3 lentiviral-transduced EC ( Fig. 6d ). Conversely, we monitored c-jun-dependent gene transcription using an AP1-responsive luciferase-based reporter, and observed that Wnt5a induction of luciferase reporter gene expression was repressed in Pdzrn3 -depleted EC and induced in Pdzrn3 lentiviral-transduced conditions ( Fig. 6e ). Taken together, these data support our hypothesis that PDZRN3 favours Dvl3 re-routing from the Wnt canonical pathway towards the PCP signalling pathway. 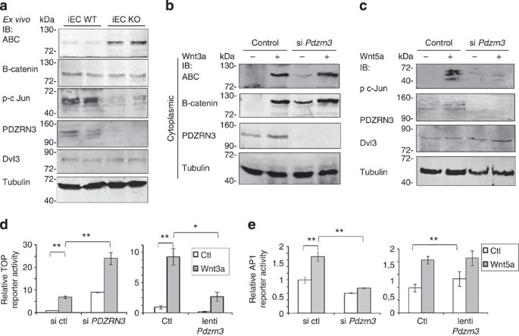Figure 6: PDZRN3 regulates the balance between non-canonical Wnt/PCP and Wnt canonical signalling in endothelial cells. (a) The Wnt canonical pathway is activated constitutively and the c-Jun-dependent/PCP pathway repressed in lung lysates from P7 mice, whenPdzrn3was silenced in endothelial cells (iEC KO) compared with lysates from control littermate mice (iEC WT) as indicated by anti-active β-catenin (ABC) and anti p–c Jun immunoblot analysis. PDZRN3 expression was evaluated. Normalization was done using the expression of α-tubulin. (b) siRNA depletion ofPdzrn3enhanced the accumulation of cytoplasmic β-catenin in HUVEC after treatment with Wnt3a CM; quantification of cytoplasmic β-catenin and ABC are normalized with cytoplasmic α-tubulin after cell fractionation. (c) The phosphorylation of c-Jun in HUVEC is indicative of activation of the PCP pathway, as a 30-min incubation with Wnt5a CM activates phosphorylation of c-Jun. Depletion ofPdzrn3blocks Wnt-mediated phosphorylation of c-Jun; quantification of c-Jun was normalized with α-tubulin. (d) Depletion ofPdzrn3(siPdzrn3) increases the activation of the TOP luciferase reporter system while lentivirusPdzrn3 (lentiPdzrn3) transduction blocks the activation of a Lef/Tcf luciferase reporter system (top reporter) after incubation with Wnt3a CM in HUVEC; experiments were performed in triplicate, error bars denote s.d.,n=3. Unpairedt-test on the average values obtained in three independent experiments. (e) Depletion ofPdzrn3(siPdzrn3) blocks activation of the AP1 luciferase reporter system after incubation with Wnt5a CM while lentivirusPdzrn3 (lentiPdzrn3) transduction activates the AP1 luciferase reporter moderately in HUVEC; experiments were performed in triplicate, error bars denote s.d.,n=3. *<0.05; **<0.01. Unpairedt-test on the average values obtained in three independent experiments. Figure 6: PDZRN3 regulates the balance between non-canonical Wnt/PCP and Wnt canonical signalling in endothelial cells. ( a ) The Wnt canonical pathway is activated constitutively and the c-Jun-dependent/PCP pathway repressed in lung lysates from P7 mice, when Pdzrn3 was silenced in endothelial cells (iEC KO) compared with lysates from control littermate mice (iEC WT) as indicated by anti-active β-catenin (ABC) and anti p–c Jun immunoblot analysis. PDZRN3 expression was evaluated. Normalization was done using the expression of α-tubulin. ( b ) siRNA depletion of Pdzrn3 enhanced the accumulation of cytoplasmic β-catenin in HUVEC after treatment with Wnt3a CM; quantification of cytoplasmic β-catenin and ABC are normalized with cytoplasmic α-tubulin after cell fractionation. ( c ) The phosphorylation of c-Jun in HUVEC is indicative of activation of the PCP pathway, as a 30-min incubation with Wnt5a CM activates phosphorylation of c-Jun. Depletion of Pdzrn3 blocks Wnt-mediated phosphorylation of c-Jun; quantification of c-Jun was normalized with α-tubulin. ( d ) Depletion of Pdzrn3 (si Pdzrn3 ) increases the activation of the TOP luciferase reporter system while lentivirus Pdzrn3 ( lenti Pdzrn3 ) transduction blocks the activation of a Lef/Tcf luciferase reporter system (top reporter) after incubation with Wnt3a CM in HUVEC; experiments were performed in triplicate, error bars denote s.d., n =3. Unpaired t -test on the average values obtained in three independent experiments. ( e ) Depletion of Pdzrn3 (si Pdzrn3 ) blocks activation of the AP1 luciferase reporter system after incubation with Wnt5a CM while lentivirus Pdzrn3 ( lenti Pdzrn3 ) transduction activates the AP1 luciferase reporter moderately in HUVEC; experiments were performed in triplicate, error bars denote s.d., n =3. *<0.05; **<0.01. Unpaired t -test on the average values obtained in three independent experiments. Full size image Endocytosis blockade delays endothelial sprouting Next, we asked whether PDZRN3-induced endocytosis is a mechanism that drives angiogenic morphogenetic events. We tested endocytosis blockade for its effect in vivo and ex vivo on sprouting endothelial cells. Intravitreal injection of dynasore or vehicle was performed in P3 neonatal pups to compare the extent of primary plexus at P5 in the control eye, and in the dynasore-injected eye of the same animal ( Fig. 7a ). Radial extension of the primary plexus in dynasore-injected eyes was significantly reduced and vessel regression was greater, demonstrated by an increase in the number of empty collagen IV sleeves without ECs, as compared with those injected with vehicle only ( Fig. 7a ). Similar results were obtained when dynasore was added ex vivo to mouse aortic ring cultures. Aortic rings were obtained from either P7 Pdzrn3 iECKO or Pdzrn3 iECWT neonatal pups. Pdzrn 3 iECKO and Pdzrn 3 iECWT treatment with dynasore led to the formation of fewer sprouts compared with Pdzrn 3 iECWT control conditions ( Fig. 7b ). Interestingly, incubation of the Pdzrn3 iECKO aortic rings with Pdzrn3 lentivirus restored their ability to form sprouts ( Fig. 7b ). We then examined whether impairment of endocytosis could impair Wnt signalling by western blot, using retina lysates. At P5, Pdzrn3 iECKO versus Pdzrn3 IECWT induced repression of p–c-jun and an increase of ABC expression ( Fig. 7c ), while intravitreal injection of dynasore decreased p–c jun level but did not affect ABC expression, suggesting that dynasore treatment partially mimics the Pdzrn3- deletion phenotype ( Fig. 7d ). We cannot exclude the possibility that the vascular morphogenetic impairment under dynasore treatment might reflect an accumulative effect on targets other than endothelial cells, such as myeloid cells. 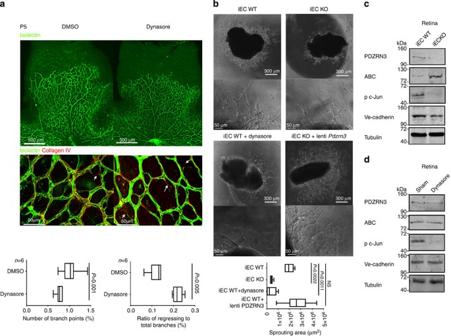Figure 7: Endocytosis is essential for activation of the PCP pathway and stability of vessels during retinal vascularization. (a) Blockade of endocytosis by dynasore intraocular injection at P3 induces retinal vasculature regression quantified at P5. The number of branch points after isolectin fluorescein isothiocyanate (FITC) staining, in the superficial plexus was decreased and capillary regression was increased in retinas injected with dynasore when compared with retinas injected with DMSO (control), as quantified by the ratio of collagen IV-positive/isolectin FITC-negative branches to total branches.n=6 DMSO injected;n=6 dynasore injected. Unpairedt-test. Scale bars, 100 μm. (b) Aortic rings were implanted in Matrigel and the area of sprouting was quantified 72 h after plating. Aortic rings from P7Pdzrn3iECKO(iEC KO) mice produce significantly smaller and less-organized sprouts, as compared with aortic rings fromPdzrn3iECWT(iEC WT) mice. Treatment of wild-type rings with dynasore reduced the number and length of sprouts while treatment of iEC KO rings withPdzrn3lentivirus (lentiPdzrn3) restores their ability to form longer sprouts;n=7 iEC KO;n=7 iEC WT, sprouting surface area was measured per aorta. Unpairedt-test. Scale bars, 50 μm. (c) At P5, the Wnt canonical pathway is activated constitutively and the c-Jun-dependent PCP pathway repressed in iEC KO retina compared with iEC WT retina, as indicated by anti-active β-catenin (ABC) and anti p–c Jun immunoblot analysis in retina lysates. (d) The level of the active form of c-Jun is downregulated at P5 by blockade of endocytosis by intraocular injection of dynasore at P3, indicating that endocytosis is an important step for activation of the planar cell polarity signalling during retinal vascularization. The level of p–c-Jun was normalized using tubulin. Expression of ABC and PDZRN3 was unchanged under dynasore treatment in contrast to that inPdzrn3deletion (iEC KO versus iEC WT) conditions. NS, not significant. Figure 7: Endocytosis is essential for activation of the PCP pathway and stability of vessels during retinal vascularization. ( a ) Blockade of endocytosis by dynasore intraocular injection at P3 induces retinal vasculature regression quantified at P5. The number of branch points after isolectin fluorescein isothiocyanate (FITC) staining, in the superficial plexus was decreased and capillary regression was increased in retinas injected with dynasore when compared with retinas injected with DMSO (control), as quantified by the ratio of collagen IV-positive/isolectin FITC-negative branches to total branches. n =6 DMSO injected; n =6 dynasore injected. Unpaired t -test. Scale bars, 100 μm. ( b ) Aortic rings were implanted in Matrigel and the area of sprouting was quantified 72 h after plating. Aortic rings from P7 Pdzrn3 iECKO (iEC KO) mice produce significantly smaller and less-organized sprouts, as compared with aortic rings from Pdzrn3 iECWT (iEC WT) mice. Treatment of wild-type rings with dynasore reduced the number and length of sprouts while treatment of iEC KO rings with Pdzrn3 lentivirus (lenti Pdzrn3 ) restores their ability to form longer sprouts; n =7 iEC KO; n =7 iEC WT, sprouting surface area was measured per aorta. Unpaired t -test. Scale bars, 50 μm. ( c ) At P5, the Wnt canonical pathway is activated constitutively and the c-Jun-dependent PCP pathway repressed in iEC KO retina compared with iEC WT retina, as indicated by anti-active β-catenin (ABC) and anti p–c Jun immunoblot analysis in retina lysates. ( d ) The level of the active form of c-Jun is downregulated at P5 by blockade of endocytosis by intraocular injection of dynasore at P3, indicating that endocytosis is an important step for activation of the planar cell polarity signalling during retinal vascularization. The level of p–c-Jun was normalized using tubulin. Expression of ABC and PDZRN3 was unchanged under dynasore treatment in contrast to that in Pdzrn3 deletion (iEC KO versus iEC WT) conditions. NS, not significant. Full size image Understanding the molecular mechanisms required for coordinating and orienting cell movements to shape vascular networks in a precise and tightly regulated pattern, is an important question in developmental biology. In this study, we used mouse loss-of-function experiments to demonstrate that the loss of E3 ubiquitin ligase Pdzrn3 activity leads to disorganization of the vascular vitelline network during embryogenesis and defects in retinal vascular branching. We have also identified Dvl ubiquitinylation as a physiological target of PDZRN3 signalling, as it is strongly reduced in the absence of Pdzrn3 in vivo and in vitro . We further demonstrate an important and unexpected role for PDZRN3, inducing PCP signalling and directing endothelial cell movements in an autonomous Fzd/Dvl-dependent manner. We then designed an in vivo study, to conditionally block Pdzrn3 expression within a narrow time window, when earlier vasculogenesis would not be affected. We induced Pdzrn3 excision after the formation of the primary vascular plexus, by injection of tamoxifen in pregnant mice at E7.5 and 8.5. By E9.5, vascular remodelling has already started in the yolk sac with large vitelline vessels and at E10.5, an intricate, orderly arrangement of large vitelline arteries and veins branching in a fractal pattern to smaller vessels can be seen. Deletion of Pdzrn3 did not impair vitelline vessel formation, but did effect the pattern of hierarchically organized, vitelline vessel architecture throughout the yolk sac. At E10.5, the mutant vascular network degenerated with numerous small disorganized vitelline vessels evenly distributed throughout the yolk sac. Moreover, embryonic vessels did not invade into the labyrinth placenta layer. Importantly, we reported that deletion with Ubc-cre reporter lines induced a more severe phenotype than the one induced with the Pdgf-cre reporter line. These differences may be due to differences in efficiency of the cre recombinase expressed in different cell lineages [33] . Moreover, phenotypic differences may be linked to a non-endothelial role of Pdzrn3 , as Pdzrn3 expression is not restricted to endothelial cells [22] . On the basis of this data, mutant embryos may die from failure to establish a functional placenta, which is required for embryo nutrition. The identification of PDZRN3 as a physiological target of Wnt signalling is consistent with previous loss-of-function analyses of Wnt signalling components in mice, reporting their involvement in different steps of placental development [34] , [35] , [36] , [37] . Interestingly, embryos deficient in Wnt2 and fzd5 share similar vascular defects . Wnt2 mutants have poorly developed labyrinth layers with reduced fetal vasculature [38] , while fzd5 -deficient embryos die in utero with early defects in the yolk sac, and placental angiogenesis with degeneration of large vitelline vessels [39] . Recently, GCM1, a key transcription factor involved in placental branching morphogenesis, was identified as a novel target of Wnt-β-catenin signalling. Its expression was decreased in BCL9-like , fzd5 and R-spondin3 -deficient mice, which all display placental defects [40] . To confirm a functional role of PDZRN3 in angiogenesis, we specifically deleted Pdzrn3 in EC using a Pdgf icre mutant. Mutants had an increase in vascular regression/remodelling of the superficial plexus, but no effect on tip cells, and a planar misorientation of the intermediate plexus in the plane orthogonal to the axis of the apical plexus, which leads to an incomplete and disorganized deep plexus. The Wnt signalling components and canonical signalling pathway have been involved in the control of hyaloid regression and primary plexus extension [5] , [6] , [10] , [41] , [42] . Recently, Wnt non-canonical signalling was shown to control the deeper, retinal layer branching. Stefater et al. [43] have shown that resident myeloid cells, via Wnt5a-dependent non-canonical signalling, can secrete sFlt1 to regulate vascular endothelial growth factor-stimulated angiogenesis. Here, we propose a novel, autonomous role of Wnt non-canonical signalling to regulate endothelial cell morphogenetic movements mainly for deeper plexus architecture. Interestingly, hyaloid vasculature and retina vasculature development could be regulated by common pathways such as the hypoxia-response pathway, which upregulates vascular endothelial growth factor-A expression [44] , [45] . An elegant paper by Rao et al. [46] reported a light-response pathway involved in the regulation of both hyaloid regression and postnatal retinal vascular development. In the current study by P14–P21 stages, hyaloid vasculature had almost completely regressed in both Pdzrn3 mutants and control littermates, while it was reported that defects in the Wnt signalling pathway may be responsible for abnormalities in hyaloid vessel regression [47] , [48] . Moreover, western blot analysis of PZRN3 expression during retinal vascularization, showed that its expression peaked at P12 after birth suggesting a late role for Pdzrn3 in retina vasculature while hyaloid regression was proposed to be temporarily regulated, with a peak around P5 [49] . Further analysis will be required to analyse the impact of Pdzrn3 deletion on hyaloid vascularization, as some of the changes observed in retinal vessels may be an indirect consequence of what happens to the hyaloid vessels. These in vivo data demonstrate that PDZRN3 signalling is required for the oriented branching architecture in vessels. Vascular maturation is a tightly regulated process, controlled by a balance of angiogenic signalling. Several recent reports have involved Wnt PCP in vascular morphogenesis [3] , [4] , [50] . Wnt PCP signalling controls large mechanisms such as, cells migration, axonal guidance, asymmetric cell division, hair or cilia orientation [12] , [14] , [51] as well as mammalian wound healing repair [52] . Manifestation of planar polarity features depends on tissue context, and as such we sought to examine the role of the PCP pathway in control of endothelial cell migration and polarity and in fine vessel morphogenesis. In vertebrate, the PCP pathway was shown to require a core of conserved proteins, including Frizzled receptors, Dvl 1/2/3, prickle1/2, diversin, Celsr1/2/3, Vangl2 and Daam1 [4] , [17] . Here, we identified Pdzrn3 as a novel PCP gene required for EC directional migration, using loss- and gain-of-function approaches in in vitro and ex vivo models. It is not yet clear how Wnt activates the PCP pathway after binding to the Fzd receptor, to impart information to EC during vascular remodelling. Fzd4 has attracted considerable attention, owing to its major role in retinal vascular plexus formation, through Wnt canonical signalling involving the receptor complex Tetraspanin-12 and LRP5 [6] , [53] . We recently reported that Fzd4 was also involved in the Wnt/PCP pathway and proposed its role in vascular morphogenesis in fzd4 KO mice [21] . Endocytic mechanisms have emerged to control either β-catenin Wnt-dependent signalling [54] , [55] , [56] or PCP signalling [27] , [30] , [57] . Importantly, endothelial cell depletion of Pdzrn3 modified the Wnt canonical versus non-canonical balance, as we found an ABC accumulation, coupled with a blockade of c-jun phosphorylation, in mutant versus control EC ex vivo and in vitro under Wnt5a stimulation. Similarly, it has been reported that Wnt5a signals through the receptor Ror2 to inhibit the β-catenin-dependent canonical Wnt signalling pathway and activate c-Jun N-terminal kinase in vitro [58] , [59] . Our demonstration that Dvl ubiquitinylation is a consequence of PDZRN3 activity, raises the possibility that the ubiquitinylated form of Dvl could be a molecular switch to specify non-canonical versus canonical functionality. However, we cannot exclude the possibility that PDZRN3 may have other still unknown substrates, which may participate in the vascular function of PDZRN3. This, then raises the possibility that part of the vascular phenotype induced under Pdzrn3 depletion may be independent of Dvl3 trafficking. It has been proposed that Wnt responsiveness is controlled by Fzd receptor levels at the cell surface via interplay between E3 ubiquitin and deubiquitine ligase [60] , [61] . Here we proposed that Dvl3-K63 polyubiquitnation could act as a cargo selection signal required to induce Fzd/Dvl complex internalization and activation of the Wnt/PCP signalling. Indeed, we report that PDZRN3 would preferentially add a K63 ubiquitin chain to Dvl3 versus K48 ubiquitin. A recent study combining genetic and quantitative proteomic approaches proposed that K63 Ub linkages is a non-degratative form of ubiquitination [62] and as such, could allow various proteasome-independent biological outcomes. For example, in a yeast model K63 ubiquitination is involved in DNA repair [63] ; and parkin-mediated K63 ubiquitination is involved in NFκB signalling [64] . As it was proposed that the routing of receptor in intracellular organelles could be an active process for signalling transduction [65] , here we provide evidence that internalization of active Fzd receptor is required for signal transduction, bringing active Fzd/Dvl complex to the intracellular compartment. Given its expression in distinct tissues, and the presence of PDZ domains that mediate protein clustering to regulate the signalling network, this indicates a broader role of PDZRN3. As a large number of cancers have been linked to deregulation of the Wnt pathway, we searched for PDZRN3 expression in high-throughput cancer profiling databases. In a human breast cancer microarray database, PDZRN3 was co-expressed with other Wnt genes such as DKK3, TCF4, netrin receptor Unc5B that is involved in EC guidance [66] and Col4A1 that is associated with autosomal-dominant hereditary angiopathy [67] (Oncomine, Compendia Bioscence, Ann Arbor, MI, USA). In a multi-cancer database, PDZRN3 expression was linked with a large number of EC markers, suggesting that PDZRN3 could be a novel Wnt signalling regulator in human cancer pathologies linked to vascular disorders. This study provides a novel molecular partner that could fine-tune Wnt complex signalling pathways to control of EC behaviour. In collectively regulating EC migration and polarity, PDZRN3 induces PCP signalling, which is critical for vascular morphogenesis. Yeast two-hybrid experiment mDvl3 lacking the DIX domain [21] was subcloned into pGBTK7 in-frame with the DNA-binding domain of galactosidase-4 (GAL4). Yeast two-hybrid screening and assays were performed as described in the Clontech protocol (MatchMaker GAL4 Two-Hybrid Sstem3, Clontech, K1612-1). AH109 cells expressing GAL4–Dvl3ΔDIX were combined with Y187 cells expressing the mouse E11 embryo complementary DNA (cDNA) library (Clontech, 638868). The mating mixture was plated on SD/ −TRY, −LEU, −HIS, −ADE, X-α-gal plates. From colonies obtained after transformation, >500 colonies tested were His positive/MEL1 positive. The library plasmids from those colonies were rescued, amplified by PCR and sequenced. Expression constructs mDvl3, Dvl3ΔDIX and Dvl3ΔPDZ cDNA sequences [21] were PCR amplified and subcloned in-frame in pcDNA3.1-myc his. Vector coding for Fzd4-HA was provided by Dr Tomas Kirchausen [30] and for Fzd4-GFP by Dr M. Montcouquiol. From Human PDZRN3 cDNA provided by Dr Makoto Inui [22] ,the full sequence and the sequence of PDZRN3, excluding the PDZ-binding motif TTV, were PCR amplified and subcloned in-frame into the pcDNA3.1-V5-His plasmid (Invitrogen), to generate PDZRN3-V5 and PDZRN3ΔPDZB-V5. Dvl3-green [21] , and PDZRN3-V5 sequence were subcloned into the lentiviral vector pRRLsin-MND-MCS-WPRE. Lentivirus preparations were produced at the Bordeaux 2 lentivirus platform. Generation of conditional Pdznr3 knockout mice All mice used in this study were bred and maintained at the institute. This study was conducted in accordance with both Univ. Bordeaux2 institutional committee guidelines (committee CEEA50) and those in force in the European community for experimental animal use (L358-86/609/EEC). Floxed Pdznr3 mice (stock 01750, Riken institute) were generated by Dr Y. Saga (National Institute of Genetics, Japan). The neomycin cassette was subsequently removed by flippase-mediated recombination by breeding with Flp mice. Floxed Pdzrn3 (PDZRN3 fl/+ ) mice were subsequently backcrossed on C57BL6/J background. Interbred, homozygous Pdzrn3 fl/fl mice exhibit apparently normal development, and are viable and fertile. Two lines of Cre mice, Ubc creERT2 (B6;129S-Tg(UBC-cre/ERT2)1Ejb/J, Jackson Lab) and PDGFb icre [68] transgenics were bred with Pdzrn3 fl/fl females to generate Pdzrn3 fl/fl ; Ubc creERT and Pdzrn3 fl/fl ; Pdgf PDGFb icre or to simplify Pdzrn3 iECKO (iEC KO), respectively. Cre-negative littermates were used as controls. To verify the efficiency of Cre recombination, Cre mice were mated with the reporter transgenic line mTmG ((ROSA)26Sor tm4(ACTB-tdTomato,-EGFP)Luo /J, Jackson Lab). For yolk sac vascularization analysis, gene inactivation was induced by tamoxifen injection (100 μl of a 10-mg ml −1 solution, corn oil) intraperitoneally in a pregnant mother daily from day 7.5 to day 9.5 or from day 10.5 to day 12.5, and pups were analysed, respectively, starting from day 10.5 and day 13.5. For pups, tamoxifen was administered by intraperitoneal injection at 50 μl of a 1-mg ml −1 solution at P1–P3. The phenotypes of the mutant mice were analysed at the reported time. Tails of pups were genotyped by PCR using the P1/P2 primer set for the wild-type allele and for the Flox allele, and the P3/P4 primer set for the KO allele: P1: 5′-cgacccacttgctccagtaaccggaaag-3′; P2: 5′-gaggctgacataattcccgatcagc-3′; P3: 5′-TCTGGCCTGTCCCATCCAGACAGCTGGAG-3′; P4: 5′-GGAGATGTTTTAATTCAAGGAGGCTATCAC-3′. For PDGF Cre-recombinase, forward primer: 5′-CCAGCCGCCGTCGCAACT-3′, and reverse primer: 5′-GCCGCCGGGATCACTCTCG-3′ (ref. 68 ) were used. Histology and immunohistochemistry For whole-mount or tissue section histologic and immunohistologic analysis, embryos and yolk sacs were fixated in 80% methanol/20% dimethylsulphoxide (DMSO) overnight, treated with 3% H 2 O 2 for 5 h to block endogenous peroxidases and then rehydrated in 50% methanol/50% phosphate-buffered saline (PBS) for analysis. Brains from embryos (E14.5) were fixed in paraformaldehyde (PFA) 4%-PBS, frozen in OCT and cryosectioned. For en face aorta staining, aorta were removed from P7 pups and fixed in PFA 4%-PBS for 30 min. Placentas were fixed in PFA 4%-PBS, then paraffin embedded and sections were stained with haematoxylin/eosin for morphologic evaluation. Briefly, immunohistochemical staining was performed in PBS supplemented with 1% donkey serum with the following antibodies: anti-CD31 (BMA Pharmingen, T-2001, 1/50), anti-PDZRN3 (Santa cruz, sc-99507, 1/50). RNA preparation and quantitative PCR Mouse tissues or cells were homogenized in TRI-REAGENT (Euromedex), and RNA were extracted according to the manufacturer’s instructions and reverse transversed using the M-MLV Reverse Transcriptase (Promega). Quantitative PCR was performed on a Bio-Rad Opticon using the Sybrgreen reagent (Life Technologies). Primer sequences are as follows: mouse beta-actin forward primer (NM_007393): 5′-ATTTCTTTTGACTTGCGGGC-3′, and reverse primer: 5′-GGAGGAGCTGGAAGCAGCC-3′; mouse PDZRN3 forward primer (NM_018884.2): 5′-CTGACTCTTGTCCTGCATCGGGACTC-3′, and reverse primer: 5′-ATGGGCTCCTTGGCTGTCTTGAAAGC-3′. Human beta-actin forward primer (NM_001101): 5′-ATTTCTTTTGACTTGCGGGC-3′, and reverse primer: 5′-GGAGGAGCTGGAAGCAGCC-3′; human PDZRN3 forward primer (NM_015009.1): 5′-ATTATTGAGGTCAACGGCAG-3′, and reverse primer: 5′-AGGGCCATGATATGTTCAAAG-3′. Mouse retina analysis Mouse eyes at P0-P21 postnatal stage were dissected and stained with isolectin-B4 (Sigma, L2895, 1/100) or collagen IV (Santa Cruz, sc-113360, 1/100) in PBS supplemented with 5% bovine serum albumin. Retinal vasculatures were imaged with a fluorescent microscope (Apo-observer, Zeiss) and vascularized retinal areas quantified with axiovision software (Zeiss). The number of branch points was quantified after skeletonization (Cell profiler) in an area of 0.25 mm 2 (8 fields per retina). To assess blood vessel regression, the ratio of the number of collagen IV-positive/isolectin-negative to the total number of capillary segments was assessed (8 fields per retina). The retinal vascularization at P12 was imaged with a confocal microscope (Olympus FV 1000) and analysed using Imaris (Bitplane). The organization of the secondary plexus was analysed using ImageJ (tracking plugin) and the Chemotaxis and Migration tool (Ibidi). BrdU staining of retina was performed as described before [41] . Counts of BrdU+ nuclei on or near vessels per field were normalized to the densities of the vessels of the field. Intraocular injection was performed using the injector from World precision instruments. dynasore (0.5μl) (200 μM in 6% DMSO; 94% ethanol) was injected in one eye of the animal at the speed of 50 nl s −1 ; the other control eye was injected with a solution of 6% DMSO; 94% ethanol. Cell culture/DNA transfection and drug treatments HEK293-Tq cells (American Type Culture Collection, ATCC, CRL-1573) were cultured in Dulbecco's modified Eagle's medium supplemented with 10% fetal bovine serum (FBS) (Hyclone) and penicillin–streptomycin. HeLa (ATCC CCL-2) and MS1 (mouse pancreatic islet endothelial cell line, ATCC CRL-2279) cells were cultured in RPMI supplemented with 10% FBS and penicillin–streptomycin. HUVECs (Lonza) and human microvascular endothelial cells (Lonza) were cultured in EGM-2 media (Lonza, CC-3156) supplemented with EGM-2 Single Quots (Lonza, CC-4176). All these cells were serum starved with Dulbecco's modified Eagle's medium plus 1% FBS/0.25% bovine serum albumin. CM from Wnt3a- and Wnt5a-producing mouse L cells (respectively, ATCC CRL-2647 and CRL-2814) was harvested as described in ATCC. Cells were activated either with Wnt3a CM or with Wnt5a CM. Plasmids were transfected using jetPRIME (Polyplus) following the manufacturer’s protocol (final concentration of 1.5 μg ml −1 for HEK293 cells, 0.5 μg ml −1 for HeLa cells). SiRNA were transfected using INTERFERin (Polyplus) at a final concentration of 30 nM. The oligonucleotides used were designed by Origene for h-pdzrn3: SR307944A, SR307944B and SR307944C. Lentivirus were tranduced at a multiplicity of infection of 20. Ly.72632 (Sigma) was used at 10 μM (Sigma). dynasore (Santa Cruz) was used at 40 μM in vitro and ex vivo . In vitro assays on endothelial cells Chemotaxis assay was carried out by plating Hoechst pre-treated HUVEC cells in μ-Slide Chemotaxis two-dimensional slides (Ibidi). After 6 h, 90 μl of control CM was added to one of the chemotaxic chamber and 90 μl of Wnt5a CM (diluted 1/20) to the other chamber, creating a gradient of Wnt factors in the capillary. The capillary was then filled with fresh medium and the slide placed for 6 h under an inverted microscope (AxioObserver, Zeiss). Nuclei of each cell were tracked during time and surfaced using Imaris software (Bitplane). For 3D tubulogenesis assay, HUVECs were transduced with control or Pdzrn3- expressing lentivirus and transfected with various siRNAs and nuclei labelled by supplementation with Hoechst (5 μg ml −1 ) for 30 min. Cells were then incubated with gelatin-coated microcarrier beads (Cytodex 3; Sigma) for 5–6 h. When the cells reached confluence, equal numbers of HUVECs-coated beads were embedded in fibrin gels in a μ-slide angiogenesis plate (Ibidi). The fibrin gel was prepared by dissolving bovine fibrinogen (2.5 mg ml −1 ; Sigma) in EBM2 medium supplemented with Aprotinin (0.05 mg ml −1 ; Sigma). Clotting was induced by the addition of thrombin (1.2 U ml −1 ) (Sigma). After 60 min, control or Wnt5a-transfected human fibroblasts were plated on the top of the gel and EBM2 medium added. The formation of tube-like structures was imaged by time-lapse videomicroscopy (in fluorescence) for 12 h under an inverted microscope (AxioObserver, Zeiss), 48 h after plating for quantification. The number of sprouts per bead, length of the sprout and number of nuclei per sprout was quantified at 96 h after plating. Luciferase reporter assay Transactivation analysis of TopFlash and AP1 reporter plasmids were performed in HUVEC cells. Briefly, the cells grown in 48-well culture plates were transiently transduced at 60–70% confluence with the 8XTOPflash reporter (Nusse lab), and a β-galactosidase reporter for normalization. Cells were activated 24 h after transfection with Wnt3a, Wnt5a or control CM. Biochemistry assays For cell fractionation, cells lysates were potterized and centrifuged at 1,000 g to obtain the pellet and the supernatant. The pellet from the cell lysate was then resuspended and loaded on cushions of sucrose 40% sucrose 30%; sucrose 20%; sucrose 16%; after a 60,000 g centrifugation, the interface between the sucrose 30% and sucrose 20% phases was collected and resuspended; finally after a spinning at 100,000, the pellet obtained corresponded to the early endosome. The supernatant from the cell lysate was centrifuged at 100,000 g and the pellet obtained was resuspended in the TRIS buffer+1% triton and spinned again for 10 min at 13,000 g . The supernatant was then collected and identified as the membrane fraction. For ubiquitinylation assay, cells were transfected with the following vectors: pRK5-HA-UB-wt, pRK5-HA-UB K48only , which codes for lysine 48-only-ubiquitin or prK5-HA-UB K63only , which codes for lysine-63-only ubiquitin (Addgene). HEK293 were co-transfected with Dvl3-myc (0.5 μg ml −1 ), one of the ubiquitin-coding plasmids (0.5 μg ml −1 ) and PDZRN3-V5 or an empty control plasmid (0.5 μg ml −1 ). For immunoprecipitation, lysates were incubated with primary antibody at +4 °C, followed by incubation with protein G-Sepharose slurry. Immunoprecipitation was carried out using the following antibodies at 2 μg for 500 μg of protein lysate: anti Dvl3 (Santa Cruz, sc 8027) and anti-myc (9E10, Millipore, 05–724). Proteins were then resolved by SDS–polyacrylamide gel electrophoresis and blotted with the following antibodies: anti-HA (Cell signalling, 3724, 1/1,000), anti rab 5 (Santa cruz, sc-9020, 1/1,000), anti V5 (Invitrogen, 46–0705, 1/3,000), anti-PDZRN3 (Santa Cruz, sc-99507, 1/500), anti c-JUN (Upstate, 06–225, 1/500), anti activated β-catenin (anti-ABC, clone 8E7, Millipore, 05–665, 1/1,000), anti-βcatenin (Sigma, C2206, 1/3,000), α-tubulin (Sigma, T5168, 1/5000), anti phosphorylated c-Jun (Cell signalling, 9261S, 1/500), anti-myc (9E10, Millipore, 05–724, 1/3,000), anti-GFP (Molecular probes, 11-814-460-001, 1/3,000), anti-Ve-cadherin (Santa Cruz, sc 6458, 1/1,000), anti-ubiquitin (Sigma, U5379, 1/1,000), anti-paxillin (Santa Cruz, sc-5574, 1/1,000 ) and anti-Dvl3 (Santa Cruz, sc 8027, 1/500). Binding of antibodies to the blots was detected using Odyssey Infrared Imaging System (LI-COR Biosciences). Uncropped scans of all western blots are presented in Supplementary Fig. 5 . Immunocytochemistry Immunofluorescence analyses were realized on HeLa or HUVECs cells. The cells were fixed in formalin 4% and stained with anti-HA (Cell signalling, 3724, 1/200), anti rab 5 (Santa cruz, sc-9020, 1/100), anti V5 (Invitrogen, 46–0705, 1/200), anti-myc (Millipore, 05–724, 1/200) and anti-ubiquitin (Sigma U5379, 1/100). Cells were imaged using a fluorescent microscope (AxioObserver, Zeiss) and analysed using Axiovision imaging software (Zeiss). For co-localization studies, cells were analysed with a confocal microscope (Olympus FV 1000). Visualization was obtained after digitized image multichannel deconvolution by Autodeblur (Media Cybernetics Inc., MD, USA) and 3D projections were digitally reconstituted from stacks of confocal optical slices by Imaris software (Bitplane) (Bitplane AG, Zurich, Swizerland). Aortic endothelial cell-sprouting assay Thoracic aorta were removed from mice P7 (males) and cut into 1-mm rings. The aortic rings were embedded in growth factor-reduced Matrigel (Becton Dickinson) on a μ-slide angiogenesis plate (Ibidi), incubated in EBM2 medium for 72 h and imaged using an Olympus inverted microscope after incorporation of Hoechst (5 μg ml −1 in medium for 30 min). The aorta rings were transduced with Pdzrn3 lentivirus or control lentivirus mixed in matrigel (10 6 particles per 100 μl of gel). The sprouting area was then quantified after surfacing using Imaris (Bitplane). Isolation of primary endothelial cells from mouse tissues Lungs were removed in PBS-containing CaCl2 and MgCl2 (Gibco), and endothelial cells were isolated after incubation with anti-CD31 (Pharmingen) and anti-endoglin (Santa Cruz) antibodies using microbeads (Miltenyi) as reported [21] . Statistical analysis Results were expressed as mean±s.d. or mean±min to max. All analyses were performed with appropriate software (Graphpad PRISM). Comparison of continuous variables between two groups was performed by a one-way analysis of variance and subsequently, if statistical significance was observed, by an unpaired t- test. A value of P <0.05 was considered to be statistically significant. How to cite this article: Sewduth, R. N. et al. The ubiquitin ligase PDZRN3 is required for vascular morphogenesis through Wnt/planar cell polarity signalling. Nat. Commun. 5:4832 doi: 10.1038/ncomms5832 (2014).